Observation of monolayer valence band spin-orbit effect and induced quantum well states in MoX2 Transition metal dichalcogenides have attracted much attention recently due to their potential applications in spintronics and photonics because of the indirect to direct band gap transition and the emergence of the spin-valley coupling phenomenon upon moving from the bulk to monolayer limit. Here, we report high-resolution angle-resolved photoemission spectroscopy on MoSe 2 single crystals and monolayer films of MoS 2 grown on highly ordered pyrolytic graphite substrate. Our experimental results resolve the Fermi surface trigonal warping of bulk MoSe 2 , and provide evidence for the critically important spin-orbit split valence bands of monolayer MoS 2 . Moreover, we systematically image the formation of quantum well states on the surfaces of these materials, and present a theoretical model to account for these experimental observations. Our findings provide important insights into future applications of transition metal dichalcogenides in nanoelectronics, spintronics and photonics devices as they critically depend on the spin-orbit physics of these materials. In the recent years, with the discovery of graphene [1] , [2] and topological insulators [3] , [4] , [5] , [6] , [7] , [8] , there has been an outburst of research activities to understand the physical properties of two-dimensional (2D) materials and their applications to optoelectronics and spintronics. One family of 2D materials that has recently attracted much attention is transition metal dichalcogenides (TMDCs) such as monolayers and few-layers of MX 2 (M=Mo, W and X=S, Se) [9] , [10] . These materials are easy to exfoliate and fabricate [11] , [12] , and have band gaps comparable in size to that of silicon (1.1–1.4 eV in bulk and 1.5–1.9 eV in monolayers) with the predicted property of transitioning from an indirect to a direct one upon reduction in size from bulk to monolayer [9] , [13] , [14] , [15] , [16] , [17] , [18] , [19] , making them remarkably suitable for potential use in electronics applications such as thin film transistors [20] . More excitingly, it has been predicted that the exotic spin-valley coupling phenomenon occurs in monolayers of TMDCs, thus making them appropriate for spintronics and valleytronics devices [21] , [22] , [23] , [24] . Nevertheless, even though many recent studies have examined the possibility of using TMDCs in single-layer transistors [25] , [26] , [27] , [28] , and have investigated their optical properties and potential use in optoelectronics [18] , [19] , [23] , [29] , [30] , [31] , [32] , surprisingly there has only been extremely limited experimental work on uncovering the key aspects of the electronic band structures of bulk, few-layers and monolayers of these materials and their modification under external effects such as doping, surface deposition or heterostructuring. The few existing momentum-resolved spectroscopic studies on these materials also lack the resolution and depth to highlight the important features of their band structures [33] , [34] , [35] , [36] , [37] . For instance, only recently, using micro-angle-resolved photoemission spectroscopy (ARPES), the evolution of the valence band at the corner of the Brillouin zone (BZ) from higher to lower binding energies upon reducing the number of layers to monolayer has been demonstrated [37] . The interest in monolayers of the MX 2 series lies in the emergence of the direct band gap as a consequence of the disappearance of van der Waals interlayer interactions in the monolayer limit [9] , [19] , as well as the valence band strong spin-orbit splitting because of the loss of inversion symmetry [9] , [21] , [22] , [37] . However, as films of TMDCs on typical substrates such as Si/SiO 2 grow in very small flakes of ~10 × 10 μm 2 and are usually composed of islands of variable thicknesses next to each other, tracking these two properties in a momentum-resolved manner has proven to be challenging. Furthermore, the splitting of the valence band top into two distinct degenerate bands in the bulk limit due to both strong spin-orbit coupling and interlayer hopping [38] could be of interest and has not been resolved to date. Moreover, until very recently MoS 2 has experimentally gotten the most attention among various members of the TMDCs family, such as MoSe 2 , WS 2 , and WSe 2 . This is despite the fact that the stronger spin-orbit coupling of the latter compounds make them more attractive for spintronics applications. Thus, in this work, we utilize ARPES to directly map the electronic band structure of bulk MoSe 2 across the entire BZ. We then study the evolution of its band structure upon in situ surface deposition with an alkali metal (potassium). Our results demonstrate the formation of a nearly free 2D electron gas (2DEG) within the potassium overlayers confined to the surface of MoSe 2 in the form of robust quantum well states (QWSs). This quantum confinement of potassium layers could potentially enhance the optoelectronics performance of bulk and thin films of the TMDCs and be utilized in optoelectronics applications of these materials. We also resolve the band structure of a monolayer of MoS 2 grown on highly ordered pyrolytic graphite (HOPG) substrate using the chemical vapour deposition (CVD) growth method and find evidence suggesting the existence of the split valence band induced by strong spin-orbit coupling and broken inversion symmetry. We compare our ARPES results with our first-principles theoretical calculations to gain microscopic insights on the electron behaviour in these materials, which is critically important for optimizing their potential performance in device settings. Crystal structure of MX 2 The crystal structure of MX 2 (M=Mo, W and X=S, Se) is a layered structure with layers of M atoms sandwiched between two layers of X atoms. These layers, which are held together through van der Waals forces, are shifted relative to each other in such a way that M atoms in one layer are placed directly above the X atoms in the neighbouring layers [9] , [10] , [34] . This crystal structure and the corresponding BZ are shown in Fig. 1b,c , respectively. The centre of the BZ is the Γ point, with M points the midpoints of the hexagonal BZ edges, and K points the corners of the hexagon. , and are the projection of these points onto the 2D surface BZ as illustrated in Fig. 1 c . X-ray photoemission spectroscopy measurements of the single crystals of MoSe 2 used in our studies reveal sharp peaks corresponding to Mo 3 s , 3 p and 3 d core levels, as well as those of Se 3 p and 3 d as shown in Fig. 1a , thus indicating the high quality of the studied samples. 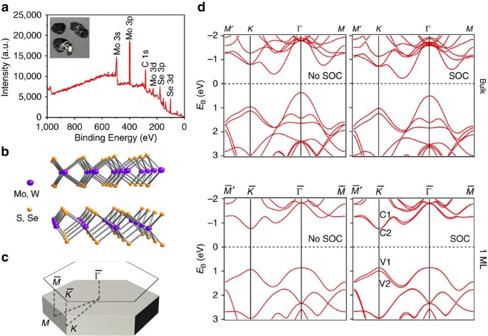Figure 1: Electronic structure of transition metal dichalcogenides (TMDCs). (a) X-ray photoemission spectroscopy measurement of the studied MoSe2crystals, showing both Mo and Se peaks. The inset shows a photograph of these crystals. (b) Three dimensional crystal structure of layered TMDCs, with the chalcogen atoms (X) in orange and the metal atoms (M) in purple. (c) The corresponding bulk and surface Brillouin zone (BZ) with the high symmetry points marked. (d) First-principles band structure calculations for bulk (top row) and monolayer (bottom row) MoS2with (right column) and without (left column) considering spin-orbit coupling, demonstrating the indirect to direct band gap transition on going to the monolayer limit and the spin-orbit splitting of the monolayer valence band. The Fermi level is indicated by the dashed lines. Figure 1: Electronic structure of transition metal dichalcogenides (TMDCs). ( a ) X-ray photoemission spectroscopy measurement of the studied MoSe 2 crystals, showing both Mo and Se peaks. The inset shows a photograph of these crystals. ( b ) Three dimensional crystal structure of layered TMDCs, with the chalcogen atoms (X) in orange and the metal atoms (M) in purple. ( c ) The corresponding bulk and surface Brillouin zone (BZ) with the high symmetry points marked. ( d ) First-principles band structure calculations for bulk (top row) and monolayer (bottom row) MoS 2 with (right column) and without (left column) considering spin-orbit coupling, demonstrating the indirect to direct band gap transition on going to the monolayer limit and the spin-orbit splitting of the monolayer valence band. The Fermi level is indicated by the dashed lines. Full size image Electronic structure of bulk MoSe 2 We start by investigating the band structure of MoSe 2 . The k – E maps of the electronic band structure measured by ARPES (left panels in Fig. 2a,b ) along the two high symmetry directions of the BZ, and , show extraordinary resemblance to the calculated bands from the first-principles calculations (right panels in Fig. 2a,b ). The ARPES measurements here were performed at a photon energy of hν =90 eV. The kinetic energy value of the Fermi level is determined by measuring that of the polycrystalline gold separately at the same photon energies and under the same experimental conditions. The valence band maximum (VBM) is found to be located at the point of the BZ at a binding energy of 1.2 eV. The valence band just below the topmost band at binding energies of ~1.7–1.9 eV, which appears clearly in our first-principle calculations, has a somewhat weaker intensity in our ARPES measurements because of matrix element effects. 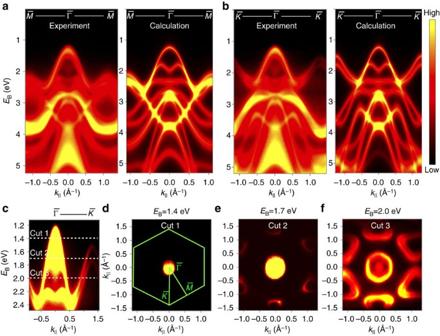Figure 2: Electronic structure and spin-degenerate bands of bulk MoSe2. (a) Angle-resolved photoemission spectroscopy (ARPES) electronic structure measurements (left panel) and first-principles calculated electronic structure (right panel) of MoSe2crystals along the high symmetry direction. (b) Same asafor measurements and calculations along the high symmetry direction. (c) Zoomed-in version of the ARPES electronic structure spectra along thedirection near the top of the valence band, highlighting the two distinct spin-degenerate bands at thepoint of the BZ. (d–f) Constant binding energy contours atEB=1.4, 1.7 and 2.0 eV, which are indicated in panelc. The green hexagon indrepresents the first BZ. The two distinct bands can also be distinguished in the contour atEB=2.0 eV inffrom the electron-like pockets around thepoints. The ARPES measurements were performed at photon energy ofhν=90 eV and temperature ofT=20 K. Figure 2: Electronic structure and spin-degenerate bands of bulk MoSe 2 . ( a ) Angle-resolved photoemission spectroscopy (ARPES) electronic structure measurements (left panel) and first-principles calculated electronic structure (right panel) of MoSe 2 crystals along the high symmetry direction . ( b ) Same as a for measurements and calculations along the high symmetry direction . ( c ) Zoomed-in version of the ARPES electronic structure spectra along the direction near the top of the valence band, highlighting the two distinct spin-degenerate bands at the point of the BZ. ( d – f ) Constant binding energy contours at E B =1.4, 1.7 and 2.0 eV, which are indicated in panel c . The green hexagon in d represents the first BZ. The two distinct bands can also be distinguished in the contour at E B =2.0 eV in f from the electron-like pockets around the points. The ARPES measurements were performed at photon energy of hν =90 eV and temperature of T =20 K. Full size image One important feature of our measurements is the unambiguous observation of the two distinct bands near the top of the valence band along the direction of the BZ. These bands are highlighted in Fig. 2 c , a zoomed-in version of the top part of the valence band along the direction, and are well in agreement with band structure calculations conducted here as well as the ones reported in earlier studies [9] , [14] , [15] (see Supplementary Note 1 and Supplementary Figs 1–3 for more details). Constant binding energy contours at representative binding energies of 1.4, 1.7 and 2.0 eV are presented in Fig. 2d–f . At E B =1.7 eV, there exists only one electron-like pocket around each of the points of the BZ (see Fig. 2e ), whereas two concentric pockets are observed at E B =2.0 eV (see Fig. 2f ), clearly resolving the two distinct bands at the BZ corners. Moreover, the hole pockets near exhibit trigonal warping effect as seen in Fig. 2e,f . This effect has been theoretically predicted in monolayer TMDCs [39] , [40] , and here we have shown that it exists in the bulk materials as well. Spin-orbit-induced splitting of the valence band in monolayer TMDCs Figure 1d shows our first-principles band structure calculations for bulk (top row) and monolayer (bottom row) MoS 2 , with (right column) and without (left column) considering spin-orbit coupling. These demonstrate the indirect to direct band gap transition on going to the monolayer limit and the spin-orbit splitting of the monolayer valence band in TMDCs. The Fermi level in these k – E maps is indicated by the dashed lines. These results are in good agreement with the previously reported first-principles calculations on this material [21] , [41] . In the next step, we turn our attention to monolayer MoS 2 on HOPG substrate. This conducting substrate was deliberately chosen to avoid the electronic charging of the film during the photoemission process. The k – E map of the electronic band structure of this sample along the high symmetry direction presented in Fig. 3a , reveals the electronic bands of monolayer MoS 2 as well as the linear π bands of graphite from the HOPG substrate at the point of the BZ. We have conducted first-principles calculations of the hybrid structure of monolayer MoS 2 and graphite ( Fig. 3b ), which indicates the general agreement with our ARPES findings. Despite the existence of the graphite’s π bands at the points, and their merging with the MoS 2 valence band around these points of the BZ, we can still resolve a large section of the MoS 2 valence band top near along the high symmetry direction , as highlighted in Fig. 3c , a zoomed-in version of Fig. 3a near the top of the valence band. 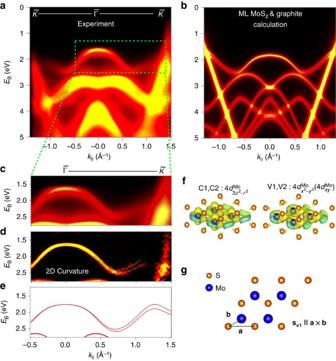Figure 3: Spin-orbit-induced splitting of the valence band in monolayer MoS2. (a) ARPES electronic structure measurements of monolayer MoS2on highly ordered pyrolytic graphite (HOPG) substrate along the high symmetry direction, showing the observation of MoS2monolayer electronic bands as well as the π bands of graphite at thepoint of the BZ. (b) First-principles calculated electronic structure measurements of monolayer MoS2accompanied by graphite along the high symmetry direction. (c) Zoomed-in version of the ARPES electronic structure spectra along thedirection. (d) 2D curvature plot of the bands near the valence band top, showing the experimental observation of the predicted spin-orbit split valence band along. The green dotted lines are guides to the eyes for these two spin-orbit split branches of the valence band. Here the ARPES measurements were performed at photon energy ofhν=110 eV and temperature ofT=200 K. (e) First-principles calculated bands near the valence band top, confirming the experimental observation of the predicted spin-orbit split valence band. (f) Charge densities of conduction and valence states at. (g) Top view of monolayer MoS2. The spin polarization of the V1 band is in the direction ofa×b, provided thatais aligned along thedirection. Figure 3: Spin-orbit-induced splitting of the valence band in monolayer MoS 2 . ( a ) ARPES electronic structure measurements of monolayer MoS 2 on highly ordered pyrolytic graphite (HOPG) substrate along the high symmetry direction , showing the observation of MoS 2 monolayer electronic bands as well as the π bands of graphite at the point of the BZ. ( b ) First-principles calculated electronic structure measurements of monolayer MoS 2 accompanied by graphite along the high symmetry direction . ( c ) Zoomed-in version of the ARPES electronic structure spectra along the direction. ( d ) 2D curvature plot of the bands near the valence band top, showing the experimental observation of the predicted spin-orbit split valence band along . The green dotted lines are guides to the eyes for these two spin-orbit split branches of the valence band. Here the ARPES measurements were performed at photon energy of hν =110 eV and temperature of T =200 K. ( e ) First-principles calculated bands near the valence band top, confirming the experimental observation of the predicted spin-orbit split valence band. ( f ) Charge densities of conduction and valence states at . ( g ) Top view of monolayer MoS 2 . The spin polarization of the V1 band is in the direction of a × b , provided that a is aligned along the direction. Full size image Moreover, we note the broadening of the valence band top along the high symmetry direction (see Fig. 3 c ). Performing 2D curvature analysis [42] of the obtained bands, we resolve two split branches of the valence band of MoS 2 along this high symmetry direction (close to the point) as shown in Fig. 3d . The green dotted lines are guides to the eyes for these two spin-orbit split branches of the valence band. This is consistent with the spin splitting scenario predicted to exist in this material, as shown by our first-principles calculations in Fig. 3e . Monolayers of TMDCs lack inversion symmetry and are non-centrosymmetric. The in-plane confinement of electron motion and high mass of the elements in these materials result in strong spin-orbit splitting of the valence band. This property makes these materials promising candidates for applications in spintronics devices [9] , [21] , [22] , [24] . Our observation here is the first momentum-resolved experimental evidence for such spin-orbit splitting. Further, spin-resolved ARPES studies are needed to identify the spin configuration of these split bands. To further demonstrate the orbital property and spin texture of monolayer MoS 2 , we calculate the charge densities and spin expectation values of the lowest two conduction states and the topmost two valence states at marked in Fig. 1d as C1, C2, V1 and V2, respectively. The charge density plots shown in Fig. 3f indicate that the dominant orbital components are Mo and Mo for C1(C2) and V1(V2), respectively. The calculated spin expectation values of states near show nearly out-of-plane spin polarization, which can be attributed to an interplay of the pure in-plane electron motion and the inversion symmetry breaking crystal potential. The out-of-plane character of Mo explains the negligible spin splitting between the C1 and C2 states. On the other hand, the calculated energy splitting between V1 and V2 states is 138 meV at , as a consequence of the prominent in-plane charge density variation of Mo orbital, which is in good agreement with previous results from density functional theory (DFT) calculations [21] , [41] . According to the calculated spin expectation values, we deploy a straightforward method to determine the spin orientation of the V1 and V2 states, which are important when considering the selection rule of polarized photon excitations. Viewing monolayer MoS 2 from top, as sulphur atoms sit on the hexagonal lattices it is alway possible to find a primitive vector connecting to adjacent sulphur atoms in the same direction as . Calling this vector a and drawing another vector b from the sulphur atom at the origin of a to the nearest Mo atom, the spin orientation of V2 is in the direction of a × b and that of V1 points to the opposite direction ( Fig. 3g ). Observation of QWSs of a nearly free 2DEG by surface deposition To study the effect of alkali metal deposition on the surface of bulk MoSe 2 , we deposit potassium (K) in situ on cleaved surfaces of crystals of this material, and track the evolution of the band structure spectra as the deposition occurs. Deposition was performed at T =60 K with an estimated deposition rate of ~0.08–0.09 Å min −1 . The total deposition time is 1 h and the nominal thickness of potassium is about 4.8–5.4 Å. 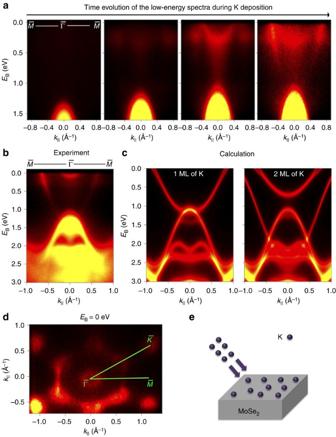Figure 4: Quantum well states (QWSs) on TMDCs through surface potassium deposition. (a) Evolution of the low-energy electronic structure of MoSe2duringin situsurface potassium deposition as measured by ARPES, showing the process of formation of in-gap quantum well states. (b) ARPES band structure spectra upon the completion of the potassium deposition process. (c) First-principles calculated band structure of one and two atomic layers of potassium on the surface of bulk MoSe2, indicating the formation of two QWSs in the ARPES measurements. (d) The Fermi surface obtained after the potassium deposition process is completed, featuring the observation of two QWSs in the form of two electron-like circular pockets around, as well as the surface states of potassium atpoints. The green lines represent theanddirections of the BZ. Here the ARPES measurements were performed at photon energy ofhν=70 eV and temperature ofT=60 K. (e) Illustration of thein situsurface potassium deposition. Figure 4a shows the evolution of the band structure k – E map along the direction of the BZ during the deposition process. We observe that the VBM at moves closer to the Fermi level by about 200 meV. We associate this shift with the formation of a conducting layer on the surface of our sample after potassium deposition. More specifically, the VBM of the MoSe 2 sample is at E B =1.0 eV, but before deposition is shifted down by about 200 meV because of the electronic charging effect (a photon-induced effect, not intrinsic to the material under study, but rather caused by the photoemission process [43] ). Next, we observe the formation of new electronic states in the band gap of MoSe 2 , extending from the Fermi level to the valence band (see middle panels in Fig. 4a ). Upon the completion of the deposition process these in-gap states are completely formed as shown in the last panel of Fig. 4a and b. Figure 4: Quantum well states (QWSs) on TMDCs through surface potassium deposition. ( a ) Evolution of the low-energy electronic structure of MoSe 2 during in situ surface potassium deposition as measured by ARPES, showing the process of formation of in-gap quantum well states. ( b ) ARPES band structure spectra upon the completion of the potassium deposition process. ( c ) First-principles calculated band structure of one and two atomic layers of potassium on the surface of bulk MoSe 2 , indicating the formation of two QWSs in the ARPES measurements. ( d ) The Fermi surface obtained after the potassium deposition process is completed, featuring the observation of two QWSs in the form of two electron-like circular pockets around , as well as the surface states of potassium at points. The green lines represent the and directions of the BZ. Here the ARPES measurements were performed at photon energy of hν =70 eV and temperature of T =60 K. ( e ) Illustration of the in situ surface potassium deposition. Full size image We note the formation of electron-like pockets on the Fermi surface after the completion of the deposition process. These pockets appear right at the points of the BZ. As the energy spacing between these pockets and the VBM (0.8 eV) is smaller than the indirect gap of MoSe 2 (~1.1 eV), we rule out the possibility of these pockets being a part of the conduction band of MoSe 2 . The resulting Fermi surface after potassium deposition shows two concentric circular-shaped pockets around the centre of the BZ, as well as the aforementioned pockets at the points ( Fig. 4d ). The circular pockets around are identified as the first and second QWSs, whereas the pockets at are possibly resulting from the surface states of potassium. We furthermore conduct first-principles calculations of potassium layers formed on the surface of bulk MoSe 2 , as shown in Fig. 4c . In the simulation, the relaxed interlayer spacing of potassium is determined to be 3.51 Å, and so the nominal thickness corresponds to 1.35–1.53 layers of freestanding K films. As an independent check of this value, we compare the ARPES spectra with DFT simulations, which gives a thickness between 1 and 2 layers, in agreement with the previous estimate (for more details see Supplementary Note 1 and Supplementary Fig. 4 ). The possibility of directly accessing the conduction band of bulk and monolayer TMDCs through intercalation and adsorption of alkali metals has been theoretically predicted [44] . Our results suggest that adsorption of alkali metals on the surface of bulk MoSe 2 results in the formation of QWSs and a nearly free 2DEG rather than electron doping and providing access to the conduction band. The splitting of the valence band along the high symmetry direction of the monolayer MoS 2 and other TMDCs, which is due to strong spin-orbit coupling (because of the high mass of the elements) and lack of inversion symmetry, has been suggested in previous theoretical studies as well as our first-principles calculations here [9] , [21] . For the bulk, this splitting is caused by the combination of interlayer interaction and spin-orbit coupling. In this case, there is no spin splitting between these two bands and they are indeed spin-degenerate (Kramers’ degeneracy) because of the presence of inversion symmetry along with time reversal symmetry. But, the strong spin-orbit coupling in TMDCs results in enhanced splitting of these spin-degenerate bands at the K point of the BZ (see Fig. 1d ) [38] . Our results resolve these two distinct bands at the corners of the BZ through ARPES measurements and theoretical first-principles calculations. Moreover, we have resolved the trigonal warping of the valence band near the point of the BZ in the bulk materials. This effect has been theoretically predicted in monolayer TMDCs and has been attributed to an anisotropic correction of order q 3 to the energy. This warping effect reflects the threefold rotational symmetry of the underlying crystal lattice [39] , [40] . From symmetry considerations, the same is expected to happen for bulk TMDCs as well, as we have shown in our measurements. Furthermore, we have provided the first momentum-resolved experimental evidence of the spin-split valence band of monolayer MoS 2 grown on HOPG substrate. However, further spin-resolved ARPES measurements are needed to confirm the spin configuration of these two split bands. According to our calculations, the maximal splitting occurs at , and is about 148 meV. The magnitude of the splitting depends on the momentum. The splitting curve rises sharply near k =0.6 Å −1 , and approaches to its maximum with a smaller slope at larger k . This momentum dependence of spin splitting can be attributed to the changes in the orbital components of the states in the valence and conduction bands (see Supplementary Note 1 and Supplementary Figs 5 and 6 for details). Recently, experimental evidence and theoretical prediction of valley confinement has been suggested in monolayer MoS 2 . Specifically, it has been suggested that the split valence band at neighbouring points of the BZ ( and ) posses opposite out-of-plane spin configurations [22] , [23] , [24] , [32] . The spin-orbit splitting observed in our study of monolayers of MoS 2 paves the way to more detailed studies of spin and valley physics in TMDCs. It also serves as a guide for spintronics and valleytronics applications of TMDCs. Our results also track the evolution of the band structure of MoSe 2 throughout the surface deposition process with an alkali metal (potassium). We note that short after the deposition process has started potassium atoms sit on the surface of MoSe 2 in a manner that results to the partial formation of the first QWS (see second panel in Fig. 4a ). Consequently, the first QWS appears in full, as shown in the third panel of Fig. 4a , and finally the second quantum well band is formed partially close to the Fermi level. The QWSs in the epitaxial potassium layers can be considered as being confined by vacuum barrier on one side and the bulk band gap of MoSe 2 on the other side [45] . When the energy of the QWS is within the bulk band gap of MoSe 2 , the state is well trapped in the epitaxial layer (for more details see Supplementary Note 1 ). In the process of surface deposition, 2D conduction channels (QWSs) emerge on the surface of the semiconducting MoSe 2 (with an indirect insulating energy gap of ~1.8 eV) and, as a consequence, the electronic behaviour of the system changes dramatically. This tunable feature can be utilized to quantitatively control the electronic properties of this quasi-2D material. Our investigation of the dynamical process in which a nearly free 2DEG is formed on TMDCs could have important implications for future optoelectronics studies and applications of TMDCs using surface manipulations by elements such as alkali metals on bulk, few-layers and monolayers of these materials. In conclusion, we have conducted detailed high-resolution ARPES and first-principles calculations studies of the electronic structure of both bulk and monolayer TMDCs. We have resolved the two distinct spin-degenerate valence bands of the bulk MoSe 2 , and have provided evidence for the spin-orbit split bands of the monolayer MoS 2 , at the corners of the BZ. We have furthermore investigated the process of the formation of QWSs on the surface of bulk MoSe 2 , and demonstrated the formation of a 2DEG on the cleaved surfaces of TMDCs. These results will be extremely valuable in designing, fabricating and optimizing these materials for future device applications. Finally, we note that after the submission of this manuscript, another group reported the splitting in the valence band of MoSe 2 monolayer and few-layers films, but neither trigonal warping effect nor QWSs on the bulk MoSe 2 were reported there [46] . Electronic structure measurements ARPES measurements were performed with incident photon energies of 35–100 eV at beamline 4.0.3 of the Advanced Light Source in the Lawrence Berkeley National Laboratory. Samples were cleaved in situ between 10 and 20 K at chamber pressure better than 5 × 10 −11 Torr resulting in shiny surfaces. Energy resolution was better than 15 meV and momentum resolution was better than 1% of the surface BZ. Sample growth and characterization To prepare MoS 2 films, molybdenum chloride (MoCl 5 ) and sulphur powder were used as precursors and the growth of monolayer films was carried out in a CVD chamber. The ultrasonicated cleaned HOPG substrates were loaded into the CVD chamber 6 cm away from the central hot zone. Argon (Ar) gas was used as carrier gas in a pressure of 3 Torr (ref. 47 ). Single crystals of MoSe 2 were grown by the chemical vapour transport method, using I 2 as the transporting agent. They were formed in silver-coloured, graphite-like, single-crystalline platelets up to 10 × 10 mm 2 in surface area and 2 mm in thickness (inset in Fig. 1 a ). X-ray photoelectron spectroscopy measurements were performed by means of Physical Electronics 5500 photoelectron spectrometer. All spectra were collected using Mg Ka X-ray operating at 300 W. The binding energy scale was calibrated by setting the main component of the C 1 s peak at 284.6 eV. First-principles calculation methods First-principles calculations of the electronic structures were performed using HGH-type pseudo-potentials [48] and a plane-wave basis set. The main programme employed was developed by the ABINIT group [49] , [50] . Spin-orbit coupling was included, where appropriate, using the relativistic local-density approximation (LDA). The experimental resolution was taken into account in the spectral simulations of Figs 2 , 3 , 4 , but the matrix element effect was not considered (see Supplementary Note 2 and Supplementary Figs 7 and 8 for more details). How to cite this article : Alidoust, N. et al. Observation of monolayer valence band spin-orbit effect and induced quantum well states in MoX 2 . Nat. Commun. 5:4673 doi: 10.1038/ncomms5673 (2014).